Injectable cryogel-based whole-cell cancer vaccines A biomaterial-based vaccination system that uses minimal extracorporeal manipulation could provide in situ enhancement of dendritic cell (DC) numbers, a physical space where DCs interface with transplanted tumour cells, and an immunogenic context. Here we encapsulate GM-CSF, serving as a DC enhancement factor, and CpG ODN, serving as a DC activating factor, into sponge-like macroporous cryogels. These cryogels are injected subcutaneously into mice to localize transplanted tumour cells and deliver immunomodulatory factors in a controlled spatio-temporal manner. These vaccines elicit local infiltrates composed of conventional and plasmacytoid DCs, with the subsequent induction of potent, durable and specific anti-tumour T-cell responses in a melanoma model. These cryogels can be delivered in a minimally invasive manner, bypass the need for genetic modification of transplanted cancer cells and provide sustained release of immunomodulators. Altogether, these findings indicate the potential for cryogels to serve as a platform for cancer cell vaccinations. The potential of the immune system to be harnessed for cancer therapy has been widely recognized for many years, beginning with Coley’s work with bacterial mixtures and more recently with T-cell co-stimulatory molecule blockade and the adoptive transfer of genetically engineered T cells [1] , [2] , [3] , [4] . Cancer vaccines have also begun to gain some traction with the FDA approval of Sipuleucel-T and are the subject of numerous ongoing clinical trials [5] . Effective cancer vaccines must first stimulate highly specific immune responses, and then bypass the ability of tumours to protect themselves from attack by cytotoxic T lymphocytes (CTLs) and antibody-dependent cell-mediated cytotoxicity. The use of whole tumour cells in cancer immunotherapy is one promising approach that obviates some of the challenges in defining specific antigens for vaccine development [6] . Whole-cell tumour vaccination offers the benefit of tumour and/or patient-specific antigen presentation to elicit immunity against a broad spectrum of tumour-associated antigens [7] . Although allogeneic cells can be used based on their relative simplicity of manufacture, autologous vaccines can be produced with patient-derived irradiated tumour cells that are genetically manipulated to release cytokines or chemokines. Two examples are GVAX and FVAX, which stimulate DCs and elicit tumour-specific immunity [8] , [9] . In GVAX, tumour cells are irradiated, engineered to overexpress granulocyte macrophage colony stimulating factor (GM-CSF) and adoptively transferred back to the patient. GM-CSF is a cytokine that plays a critical role in immunoregulation, leukocyte development, proliferation and survival, and promotes the accumulation of specialized antigen-presenting cells such as DCs through potentially multiple mechanisms including direct cellular recruitment, differentiation of precursor cell populations and changes in cell proliferation and death [10] , [11] . DCs play an important role in adaptive immunity, and adoptive transfer of immunogenic DCs loaded with tumour antigens has also been used in many cancer vaccination trials [9] , [12] . FVAX involves the engineered production of Flt3-ligand, another cytokine critical to DC function [8] . Despite the promise of whole-tumour cell vaccination, the approach typically requires substantial ex vivo genetic manipulation of tumour cells, leading to high cost and significant regulatory concerns, and the results of phase 3 trials to date have been disappointing [13] . One mechanism that may account for the limited efficacy observed in many clinical trials is the lack of co-stimulation in the setting where DCs encounter the transferred tumour cells. In vaccination more generally, adjuvants such as toll-like receptor (TLR) ligands are often used to activate the innate immune system and potentiate downstream immunity, and recently they have been added to enhance the effectiveness of whole cell tumour vaccine formulations [14] . The limited success of whole-cell vaccines may also be secondary to diffuse cellular localization and short-term survival post adoptive transfer. Poor cell localization combined with rapid cell death may lead to transient and low local GM-CSF levels, and reduce the duration of tumour antigen presentation [15] . We hypothesize that a biomaterial-based vaccination system with minimal extracorporeal manipulation can localize and maintain transferred cells to a specific microenvironment, whereby DCs can interface with tumour cells in an immunogenic context. These properties could evoke protective immunity, break tumour tolerance and elicit durable, tumour-specific immunity. To address this hypothesis, we designed tumour cell-loaded cryogel sponges that could function as an injectable vaccine platform, delivering antigen-carrying tumour cells along with GM-CSF and a specific TLR agonist, cytosine-phosphodiester-guanine oligodeoxynucleotide (CpG ODN, adjuvant), while creating a space for DC infiltration and trafficking. We have previously demonstrated that the pre-loading of tumour cells within the cryogel in vitro can improve viability and localization of transplanted cells [16] . Herein we tested the ability of the vaccine platform to coordinate the release of GM-CSF and CpG ODN, enrich for a heterogeneous network of DCs following injection, induce DC maturation by creating a potent immunogenic environment locally and evoke a strong T-effector response including CTLs [17] , [18] . Finally, to further demonstrate the ability of the vaccine to induce a potent and durable T-effector response, the vaccine was tested in a murine melanoma model commonly used as a pre-clinical system for vaccine development [19] , [20] . Cryogel characterization Injectable sponges for cell delivery were fabricated using a cryogelation technique ( Fig. 1a ), and these contained large, continuously interconnected macropores throughout the entire cryogel construct ( Fig. 1b,c ). Seeded irradiated tumour cells (3,500 rads) were homogeneously distributed in the gel pores. Cryogels were fabricated with alginate containing covalently coupled RGD peptides with the aim of enhancing tumour cell attachment through integrin binding. RGD modification led to attachment and spreading of cells after 6 h of incubation ( Fig. 1d,e , Supplementary Movie 1 ). Nanoporous hydrogels are typically brittle, but MA-alginate cryogels can undergo large levels of strain while being readily compressed to a fraction of their size and injected through a surgical needle for delivery [15] . These scaffolds quickly recover their original memorized shape once injected into the subcutaneous tissue ( Supplementary Fig. 1 ). 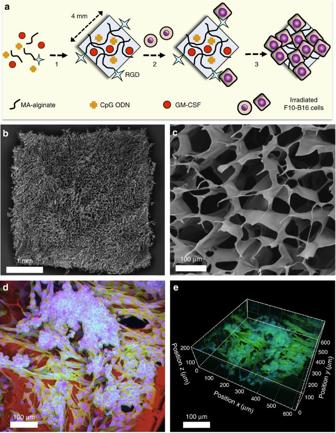Figure 1: Fabrication and imaging of irradiated tumour cell-loaded cryogel sponge vaccines. (a) Preparation of an alginate-derived active vaccine containing viable irradiated B16-F10 cells for the treatment of melanoma in syngeneic C57BL/6 mice. CpG ODN (TLR9-based immune adjuvant) and GM-CSF (cytokine adjuvant)-loaded RGD-containing alginate cryogels were prepared by a cryogelation process at subzero temperature. The gels were subsequently seeded with irradiated B16-F10 melanoma cells (depicted as round-shaped cells) and incubated for 6 h (depicted as square-shaped spread cells) before animal vaccination via subcutaneous injection. (b) SEM showing homogeneous macroporous microstructure throughout the square-shaped sponge-like gel construct. (c) SEM cross-sectional image of an alginate cryogel showing the interconnected macroporous network. (d) 2-D confocal micrograph displaying immobilization of irradiated B16-F10 cells on a typical RGD-containing cryogel after 6 h culture. Actin filaments in cells were visualized by staining with Alexa Fluor 488-phalloidin (green), cell nuclei were stained with DAPI (blue), and polymer walls were stained with polylysine-labelled rhodamine (red). (e) 3-D reconstructed confocal fluorescence micrograph of irradiated B16-F10 cells in cryogel, depicting cell adhesion, spreading and elongation after 6 h culture. Figure 1: Fabrication and imaging of irradiated tumour cell-loaded cryogel sponge vaccines. ( a ) Preparation of an alginate-derived active vaccine containing viable irradiated B16-F10 cells for the treatment of melanoma in syngeneic C57BL/6 mice. CpG ODN (TLR9-based immune adjuvant) and GM-CSF (cytokine adjuvant)-loaded RGD-containing alginate cryogels were prepared by a cryogelation process at subzero temperature. The gels were subsequently seeded with irradiated B16-F10 melanoma cells (depicted as round-shaped cells) and incubated for 6 h (depicted as square-shaped spread cells) before animal vaccination via subcutaneous injection. ( b ) SEM showing homogeneous macroporous microstructure throughout the square-shaped sponge-like gel construct. ( c ) SEM cross-sectional image of an alginate cryogel showing the interconnected macroporous network. ( d ) 2-D confocal micrograph displaying immobilization of irradiated B16-F10 cells on a typical RGD-containing cryogel after 6 h culture. Actin filaments in cells were visualized by staining with Alexa Fluor 488-phalloidin (green), cell nuclei were stained with DAPI (blue), and polymer walls were stained with polylysine-labelled rhodamine (red). ( e ) 3-D reconstructed confocal fluorescence micrograph of irradiated B16-F10 cells in cryogel, depicting cell adhesion, spreading and elongation after 6 h culture. Full size image Macroporous alginate sponges were designed to present GM-CSF and CpG ODN in a sustained and localized manner. GM-CSF was physically encapsulated (85% efficiency) into cryogels through the crosslinking process and released in a sustained manner (>80% bioactivity retention, Supplementary Fig. 2 ); the incorporation of a second immunostimulatory agent (CpG ODN) did not alter the release profile of GM-CSF ( Fig. 2a,b ), although the encapsulation efficiency was slightly lower (75%). CpG ODN was also physically immobilized and homogeneously distributed within the polymer network of alginate ( Supplementary Fig. 3 ), and the encapsulation efficiency (45%) was independent of the incorporation of GM-CSF ( Fig. 2c ). The inferior encapsulation efficiency of negatively charged CpG ODN could be attributed to a combination of its low molecular mass coupled with electrostatic repulsion to negatively charged alginate chains. Approximately 80% of the encapsulated GM-CSF and CpG ODN were released within the first 4 days, followed by a sustained release over the next month ( Fig. 2d ); these release profiles were chosen to enable diffusion of the factors through the surrounding tissue to effectively enrich and activate resident DCs over an extended time frame. 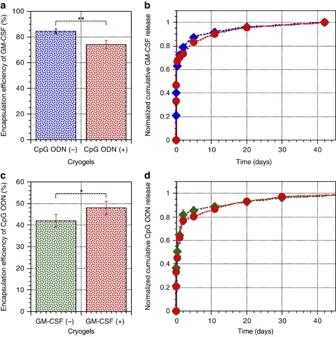Figure 2: Controlled release of biologically active immunomodulators from cryogels. (a) Encapsulation efficiency of GM-CSF (detected by ELISA) in alginate cryogels following polymerization, washing and sterilization; GM-CSF was incorporated in the presence (+) or absence (−) of CpG ODN in the cryogel. (b) Cumulative release of GM-CSF from alginate cryogels over a period of 6 weeksin vitro; blue: cryogels containing only 1.5 μg GM-CSF, red: cryogels containing 1.5 μg GM-CSF+50 μg CpG ODN. (c) Encapsulation efficiency of CpG ODN (detected by an OliGreen assay) in alginate cryogels post polymerization, washing and sterilization; CpG ODN was incorporated in the presence (+) or absence (−) of GM-CSF in the cryogel. (d) Cumulative release of CpG ODN from alginate cryogel matrices over a period of 6 weeks; green: cryogels containing only 50 μg CpG ODN, red: cryogels containing 1.5 μg GM-CSF+50 μg CpG ODN. Values represent mean and s.d. (n=5). Differences between groups were statistically significant. Data were analysed using Student’st-test, *P<0.05, **P<0.01. Figure 2: Controlled release of biologically active immunomodulators from cryogels. ( a ) Encapsulation efficiency of GM-CSF (detected by ELISA) in alginate cryogels following polymerization, washing and sterilization; GM-CSF was incorporated in the presence (+) or absence (−) of CpG ODN in the cryogel. ( b ) Cumulative release of GM-CSF from alginate cryogels over a period of 6 weeks in vitro ; blue: cryogels containing only 1.5 μg GM-CSF, red: cryogels containing 1.5 μg GM-CSF+50 μg CpG ODN. ( c ) Encapsulation efficiency of CpG ODN (detected by an OliGreen assay) in alginate cryogels post polymerization, washing and sterilization; CpG ODN was incorporated in the presence (+) or absence (−) of GM-CSF in the cryogel. ( d ) Cumulative release of CpG ODN from alginate cryogel matrices over a period of 6 weeks; green: cryogels containing only 50 μg CpG ODN, red: cryogels containing 1.5 μg GM-CSF+50 μg CpG ODN. Values represent mean and s.d. ( n =5). Differences between groups were statistically significant. Data were analysed using Student’s t -test, * P <0.05, ** P <0.01. Full size image The bioactivity of the CpG released from the cryogel vaccines was next analysed in vitro ( Fig. 3a ). Exposure of BMDCs to the cryogels did not alter CD11c expression, as expected ( Fig. 3b ). However, ∼ 60% of BMDCs exposed to CpG-loaded cryogels (group C, Fig. 3c , Supplementary Fig. 4 ) stained positively for CD86 and MHCII, similarly to the CpG ODN positive control (group D). The cells cultured with blank cryogels (group B, Fig. 3c , Supplementary Fig. 4 ) had similar cell surface expression of CD86 and MHCII as the negative control (group A, Fig. 3c , Supplementary Fig. 4 ). As activated DCs are known to secrete IL-6, IL-12 and TNF-α, the elaboration of these factors was evaluated in the context of the cryogels. Unlike GM-CSF, CpG ODN released from the cryogels induced a significant upregulation of IL-6, IL-12 and TNF-α secretion, as opposed to biomolecule-free, blank cryogels, which induced minimal cytokine production ( Fig. 3d , Supplementary Fig. 5 ). Cells in all experimental conditions exhibited high viability ( Supplementary Fig. 6 ). This set of data suggests that the released CpG ODN remains bioactive. 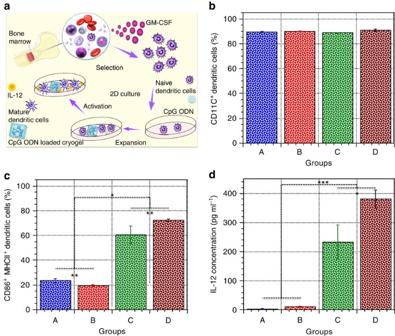Figure 3:In vitroactivation of BMDCs in response to CpG ODN-loaded cryogels. (a) Cartoon depicting the process of bone marrow cell isolation from murine tibias and femurs; the differentiation and expansion of BMDCs; and assessment of their activation in response to CpG ODN released from cryogel vaccines. BMDCs were cultured for 24 h in the following conditions: medium (A, negative control), blank cryogels/medium (B), CpG ODN loaded cryogels/medium (C), or soluble CpG ODN/medium (D, positive control). (b) Fraction of cells (detected by immunostaining in conjunction with flow cytometry) used in each condition that were CD11c+prior to stimulation. (c) Fraction of activated CD86+MHCII+BMDCs (detected by immunostaining in conjunction with flow cytometry) obtained in each condition. (d) Production of IL-12 (detected by ELISA) in culture media in response to DCs stimulated by exposure to the various conditions. Values represent mean and s.d. (n=5). Differences between groups were statistically significant. Data were analysed using Student’st-test and one-way analysis of variance (ANOVA), *P<0.05, **P<0.01, ***P<0.001. Cartoon inaadapted by permission from Macmillan Publishers Ltd: (Nature Reviews Immunology) (Holger Hackstein and Angus W. Thomson, Dendritic cells: emerging pharmacological targets of immunosuppressive drugs, 1:24-34), copyright (2004). Figure 3: In vitro activation of BMDCs in response to CpG ODN-loaded cryogels. ( a ) Cartoon depicting the process of bone marrow cell isolation from murine tibias and femurs; the differentiation and expansion of BMDCs; and assessment of their activation in response to CpG ODN released from cryogel vaccines. BMDCs were cultured for 24 h in the following conditions: medium (A, negative control), blank cryogels/medium (B), CpG ODN loaded cryogels/medium (C), or soluble CpG ODN/medium (D, positive control). ( b ) Fraction of cells (detected by immunostaining in conjunction with flow cytometry) used in each condition that were CD11c + prior to stimulation. ( c ) Fraction of activated CD86 + MHCII + BMDCs (detected by immunostaining in conjunction with flow cytometry) obtained in each condition. ( d ) Production of IL-12 (detected by ELISA) in culture media in response to DCs stimulated by exposure to the various conditions. Values represent mean and s.d. ( n =5). Differences between groups were statistically significant. Data were analysed using Student’s t -test and one-way analysis of variance (ANOVA), * P <0.05, ** P <0.01, *** P <0.001. Cartoon in a adapted by permission from Macmillan Publishers Ltd: (Nature Reviews Immunology) (Holger Hackstein and Angus W. Thomson, Dendritic cells: emerging pharmacological targets of immunosuppressive drugs, 1:24-34), copyright (2004). Full size image Immune cell recruitment and trafficking Cryogels were next analysed for their capacity to promote cellular infiltration and immune cell trafficking in situ ( Fig. 4a ). First, in an initial study blank and cell-free cryogels, and their nanoporous counterparts were surgically implanted into the subcutaneous pockets of mice (nanoporous gels must be implanted as they fracture with injection). After 4 days, blank macroporous cryogels demonstrated substantially greater cellular infiltration when compared with nanoporous hydrogels, as 6 × 10 6 cells were resident in cryogels as opposed to 0.2 × 10 6 cells in nanoporous gels ( Fig. 4b ). The interconnected macroporous architecture of cryogels is likely responsible for this increase in cellular infiltration. The ability of cryogels to selectively enrich DCs to the vaccination site was next analysed by injecting GM-CSF-loaded cryogels. A local progressive swelling at the vaccination injection site was observed within the first 2 weeks, indicative of the recruitment of immune cells ( Supplementary Fig. 7 ). Cellular examination after 4 days revealed that sponges loaded with 1.5 μg of GM-CSF led to a significant increase in the total number of cells, and more particularly infiltration by DCs ( Fig. 4c , Supplementary Fig. 8 ). Further, flow cytometry showed that GM-CSF increased the fraction of CD11b + CD11c + DCs in comparison with blank cryogels ( Fig. 4d,e ), with the double-negative cells possibly reflecting neutrophil infiltrate with some monocytes/macrophages and lymphocytes, as these characterize early wound healing and the inflammatory response that typically occurs following material implantation. Importantly, GM-CSF delivery resulted in a number of DCs residing in the biomaterial that was three times higher than the quantity typically administered with ex vivo DC manipulation protocols ( ∼ 10 6 cells). The ability of GM-CSF delivery to promote greater cellular infiltration was further demonstrated by histological analysis ( Fig. 4f,g ). Cell size, morphology, staining pattern and nuclear to cytoplasmic ratio reflect cells of varying leukocyte lineages. 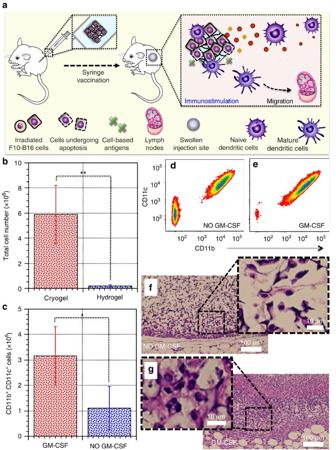Figure 4: Cryogel vaccines promote cellular infiltration and leukocyte recruitment. (a) Schematic representation displaying the subcutaneous injection of cryogel vaccines in mice using a standard hypodermic needle, resulting in local oedema and induration at the injection site, and recruitment and activation of DCs. (b) Quantification of total cellular infiltration in macroporous cryogel sponges versus conventional nanoporous hydrogels 4 days post injection. (c) Quantification of the number of CD11b+CD11c+cells infiltrating cryogels loaded with GM-CSF or blank (Control, NO GM-CSF) cryogels. (d,e) FACS analysis for CD11b+CD11c+DCs in blank (Control,d) or GM-CSF releasing cryogels (e). (f,g) H&E staining of sectioned cryogel scaffolds 4 days subsequent to subcutaneous injection in the backs of C57BL/6 J mice: blank scaffolds (f) and GM-CSF (1.5 μg)–loaded scaffolds (g). Values represent mean and s.d. (n= 5). Differences between groups were statistically significant. Data were analysed using Student’st-test, *P<0.05, **P<0.01. Figure 4: Cryogel vaccines promote cellular infiltration and leukocyte recruitment. ( a ) Schematic representation displaying the subcutaneous injection of cryogel vaccines in mice using a standard hypodermic needle, resulting in local oedema and induration at the injection site, and recruitment and activation of DCs. ( b ) Quantification of total cellular infiltration in macroporous cryogel sponges versus conventional nanoporous hydrogels 4 days post injection. ( c ) Quantification of the number of CD11b + CD11c + cells infiltrating cryogels loaded with GM-CSF or blank (Control, NO GM-CSF) cryogels. ( d , e ) FACS analysis for CD11b + CD11c + DCs in blank (Control, d ) or GM-CSF releasing cryogels ( e ). ( f , g ) H&E staining of sectioned cryogel scaffolds 4 days subsequent to subcutaneous injection in the backs of C57BL/6 J mice: blank scaffolds ( f ) and GM-CSF (1.5 μg)–loaded scaffolds ( g ). Values represent mean and s.d. ( n = 5). Differences between groups were statistically significant. Data were analysed using Student’s t -test, * P <0.05, ** P <0.01. Full size image Next, to characterize the impact of the cryogel system, we measured the magnitude and duration of the immune response resulting from both vaccination via subcutaneous injection and subsequent challenge, by the extent of DC and T-cell recruitment and immobilization. Following injection of the cryogels with or without subsequent tumour challenge, cells were isolated and analysed from the cryogels and surrounding tissues, spleen and inguinal lymph nodes (LN) to determine the overall number of cells, and the fraction of DCs and T cells ( Supplementary Fig. 9 ). The intensity of the immune response to the vaccines was reflected in the large number of cells infiltrating the vaccine site and in the expansion of cells in the LN and spleen. Particularly, an increase in the number of cells in the spleen was observed with a substantial enlargement of the organ ( Supplementary Fig. 10 ). Overall, the total number of cells was markedly increased for the vaccinated mice (with or without subsequent challenge), unlike untreated animals. Of note, the number of cells remained relatively high within the first 2 weeks following vaccination and started to noticeably drop by day 13. This trend was observed across the three investigated sites. The subpopulations of immune cells were also identified. CD11c + DCs were rapidly and significantly enriched at the vaccine site within the first 2 weeks, peaking at day 9, likely due to the high initial levels of GM-CSF at the scaffold site ( Supplementary Fig. 9 ). Later, DC numbers fell while the number of CD3 + T cells increased ( Supplementary Fig. 9 ). The accumulation of CD3 + T cells at the vaccine site peaked at day 13 and dropped sharply by day 24, possibly due to antigen clearance. Taken together these data support a model where activated DCs may home to the peripheral lymphoid organs, and interact with T cells to stimulate anti-tumour responses. Cryogel vaccines expand DC subsets and CD8 + T cells To better understand the cellular response to the cryogel vaccines, subpopulations of DCs and T-cell types at the vaccine site, draining LN and spleen were examined at the peak of infiltration for each cell type, along with cytokine expression at the vaccine site ( Fig. 5 , Supplementary Fig. 11 ). Nine days following vaccination, the number of CD11c + cells as well as the numbers of plasmacytoid and CD8 + DCs in the vaccinated groups at the implantation site, the draining LN and spleen were greater than the group with blank cryogels used as a control ( Fig. 5a–c , Supplementary Fig. 11 ). For the vaccinated groups at all of the sites examined, plasmacytoid DCs (pDCs) represented greater than 50% of all of the DCs while CD8 + DCs constituted between a quarter to a third of the remaining DCs. Taken together, these data indicate that the cryogel vaccine activates a heterogeneous network of DCs. 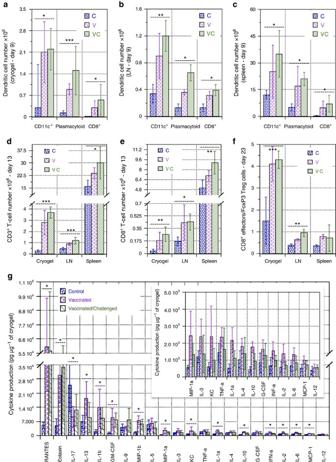Figure 5: Cryogel vaccines stimulate the recruitment and activation of innate and adaptive immune cells. Number of CD11c+DCs, pDCs and CD8+DCs at day 9 post-immunization isolated from explanted cryogel vaccines (a) regional LN (b) and spleen (c) Number of CD3+T cells (d) and CD8+T cells (e) at day 13 post-immunization isolated from explanted cryogel vaccines, LN and spleen. (f) Ratio of CD8+T cells versus FoxP3+Treg cells residing within cryogel vaccines, LN and spleen at day 23 after immunization. (g)In vivoconcentrations of the indicated mouse cytokines (detected by a Bio-Plex Pro Mouse Cytokines 23-plex Immunoassay) from explanted cryogels at day 13. The inset shows a zoomed-in view of low cytokine levels. C, V and VC groups correspond to mice injected with blank cryogels at day 0 (C), mice immunized with cryogel vaccines (containing CpG ODN, GM-CSF and irradiated B16-F10 cells) at day 0 (V), and mice immunized with cryogel vaccines at day 0+tumour challenged with live B16-F10 cells at day 6 (VC), respectively. Values ina,b,c,d,fandgrepresent mean and s.d. (n=5). Data were analysed using one-way analysis of variance (ANOVA), *P<0.05, **P<0.01, ***P<0.001 versus all other experimental conditions unless otherwise noted. Figure 5: Cryogel vaccines stimulate the recruitment and activation of innate and adaptive immune cells. Number of CD11c + DCs, pDCs and CD8 + DCs at day 9 post-immunization isolated from explanted cryogel vaccines ( a ) regional LN ( b ) and spleen ( c ) Number of CD3 + T cells ( d ) and CD8 + T cells ( e ) at day 13 post-immunization isolated from explanted cryogel vaccines, LN and spleen. ( f ) Ratio of CD8 + T cells versus FoxP3 + Treg cells residing within cryogel vaccines, LN and spleen at day 23 after immunization. ( g ) In vivo concentrations of the indicated mouse cytokines (detected by a Bio-Plex Pro Mouse Cytokines 23-plex Immunoassay) from explanted cryogels at day 13. The inset shows a zoomed-in view of low cytokine levels. C, V and VC groups correspond to mice injected with blank cryogels at day 0 (C), mice immunized with cryogel vaccines (containing CpG ODN, GM-CSF and irradiated B16-F10 cells) at day 0 (V), and mice immunized with cryogel vaccines at day 0+tumour challenged with live B16-F10 cells at day 6 (VC), respectively. Values in a , b , c , d , f and g represent mean and s.d. ( n =5). Data were analysed using one-way analysis of variance (ANOVA), * P <0.05, ** P <0.01, *** P <0.001 versus all other experimental conditions unless otherwise noted. Full size image At day 13, the number of CD3 + T lymphocytes in the cryogel sponges and the LN was greater in vaccinated mice (up to 10-fold increase at the vaccine site) when compared with non-treated animals ( Fig. 5d , Supplementary Fig. 11 ). Similarly, the number of CD8 + T cells was greater in the groups of immunized mice at the three investigated sites ( Fig. 5e , Supplementary Fig. 11 ). These data demonstrate that a strong T-effector response is triggered after vaccination, regardless of tumour challenge at day 6. On the basis of these data, the extent of regulatory T cells (Tregs) was evaluated. Tregs, identified as the FoxP3 + subset of CD4 + T cells, are known to play pivotal roles in controlling the balance between immune stimulation and suppression. No significant difference in Treg numbers with vaccination was observed; however, the number of CD8 + effectors rose in the immunized animals and the ratio of CD8 + effectors to FoxP3 + T cells at day 23 was greater in the vaccinated mice in comparison with controls at all of the investigated sites, particularly at the cryogel vaccine site ( Fig. 5f , Supplementary Fig. 11 ). Within the biomaterial, the ratio of CD8 + to FoxP3 + T cells was over 2.5 times greater than that in blank cryogels. These data suggest that the effect of immunosuppression by FoxP3 + Tregs is reduced by using cryogel vaccines that mimic local infections in contrast to the expansion of protective CD8 + T cells. In addition, at day 13, the cryogels and surrounding tissue were resected, and distinct biomarkers were measured ( Fig. 5g ). The concentration of many cytokines screened, especially RANTES, eotaxin, GM-CSF, IL-1β, IL-1α, IL-2, IL-10, IL-13, MIP-1α, MIP-1β, was greater in the tissue of the vaccinated animals compared with the control animals that received blank cryogels. In particular, the concentration of RANTES (CCL5), a cytokine known to play an active role in recruiting leukocytes into inflammatory sites, was markedly elevated and found to be at least 10-fold greater. Further, the production of a unique combination of cytokines such as eotaxin, GM-CSF and IL-1β was quantified to be over fivefold greater in experimental animals compared with controls. The upregulation of pro-inflammatory cytokines supports the notion of immune-cell activation and inflammation. Surprisingly, the local production of IL-12, TNF-α and IFN-α was not markedly upregulated after vaccination at this time point. This may be partially attributed to the specific time point analysed and likely could be enhanced if other CpG classes were utilized, although significant CD8 + T-lymphocyte immune responses were elicited. Overall, there was no statistically significant difference in cell numbers and subpopulation of immune cells between the vaccinated and vaccinated/challenged groups. Cryogel vaccines confer long-lasting protective immunity The ability of the cryogel vaccine to evoke anti-tumour immunity was then tested in a prophylactic setting using a melanoma model. We evaluated the impact of the injectable cryogel sponge that integrated and coordinated the delivery of antigen-displaying tumour cells, adjuvant and chemoattractant. Importantly, the tumour cells used as the antigen source in the cryogel were not transduced to overexpress GM-CSF, as GM-CSF was released from the cryogel itself. This immunization regimen provided a specific and markedly protective anti-tumour immunity, as up to 80% of mice survived ( Fig. 6a , Supplementary Fig. 12a ). Cryogel vaccines containing both immunostimulatory factors with autologous irradiated tumour cells elicited a more robust immunological response than cryogels containing only one of the two molecules, as indicated by survival rates ( Fig. 6a ) and tumour progression ( Fig. 6b ). Overall, the mice immunized with all of the different regimens containing the TLR-activating CpG ODN displayed a delay in tumour onset, significantly retarded tumour growth, and prolonged survival ( Fig. 6a,b ). 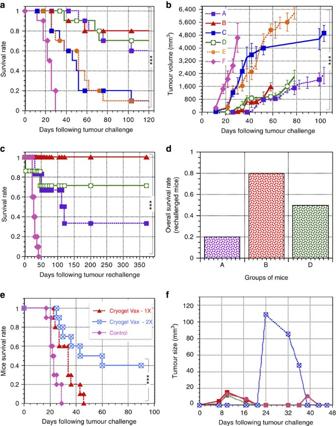Figure 6: Cryogel vaccines confer long-term prophylactic and therapeutic protection against melanoma. (a) A comparison of the survival rate in challenged C57BL/6 mice previously prophylactically vaccinated with (A) bolus vaccine injection (4 × 105irradiated B16-F10 cells+soluble 3 μg GM-CSF+soluble 100 μg CpG ODN); (B) Cryogel vaccines (2 × 2 × 105irradiated B16-F10 cells+2 × 1.5 μg GM-CSF+2 × 50 μg CpG ODN); (C) Cryogel vaccines (2 × 2 × 105irradiated B16-F10 cells+2 × 1.5 μg GM-CSF); (D) Cryogel vaccines (2 × 2 × 105irradiated B16-F10 cells+2 × 50 μg CpG ODN); (E) Blank cryogel (control; negative control); (F) naive mice (no immunization). At day 6 following immunization, C57BL/6 J mice (10 mice/group) were challenged with 105B16-F10 tumour cells and monitored for animal survival. (b) Tumour growth curve after the first tumour challenge (105cells) on prophylactically vaccinated mice. (c) A comparison of the survival rate in re-challenged mice prophylactically treated with (A) bolus injection (4 × 105irradiated B16-F10 cells+soluble 3 μg GM-CSF+soluble 100 μg CpG ODN); (B) Cryogel vaccine (2 × 2 × 105irradiated B16-F10 cells+2 × 1.5 μg GM-CSF+2 × 50 μg CpG ODN); (D) Cryogel vaccine (2 × 2 × 105irradiated B16-F10 cells+2 × 50 μg CpG ODN); and (F) naive mice (no immunization). At day 126 following immunization, C57BL/6 J mice (10 mice/group) from the first challenge study were challenged a second time with 105B16-F10 tumour cells and monitored for survival. (d) Overall survival rate after two consecutive tumour challenges in prophylactically immunized mice to evaluate long-term immunological protection in the context of melanoma. Overall survival is defined as the fraction of mice that survive both challenges. (e) A comparison of the survival of mice bearing established melanoma tumours (inoculated with 5 × 105B16-F10 cells and allowed to develop for 3 days, tumour area≥10 mm2) and therapeutically treated with cryogel vaccines (2 × 2 × 105irradiated B16-F10 cells+2 × 1.5 μg GM-CSF+2 × 50 μg CpG ODN) either once at day 3 (Cryogel Vax – 1X) or at both days 3 and 10 (Cryogel Vax – 2X), or naive mice (Control, no immunization). (f) Individual tumour growth curves for each mouse surviving tumour challenge (5 × 105cells) after a two-time treatment with cryogel vaccines at days 3 and 10. Values represent mean and s.d. (n=10 per condition) from at least two independent studies. For simplification, only Fig. 6b shows the legend but it applies also to Fig.6a, c and d. Data were analysed usingχ2-test, log-rank test (survival curves comparison), or one-way analysis of variance (ANOVA) (**P<0.01, ***P<0.001). Figure 6: Cryogel vaccines confer long-term prophylactic and therapeutic protection against melanoma. ( a ) A comparison of the survival rate in challenged C57BL/6 mice previously prophylactically vaccinated with (A) bolus vaccine injection (4 × 10 5 irradiated B16-F10 cells+soluble 3 μg GM-CSF+soluble 100 μg CpG ODN); (B) Cryogel vaccines (2 × 2 × 10 5 irradiated B16-F10 cells+2 × 1.5 μg GM-CSF+2 × 50 μg CpG ODN); (C) Cryogel vaccines (2 × 2 × 10 5 irradiated B16-F10 cells+2 × 1.5 μg GM-CSF); ( D ) Cryogel vaccines (2 × 2 × 10 5 irradiated B16-F10 cells+2 × 50 μg CpG ODN); (E) Blank cryogel (control; negative control); (F) naive mice (no immunization). At day 6 following immunization, C57BL/6 J mice (10 mice/group) were challenged with 10 5 B16-F10 tumour cells and monitored for animal survival. ( b ) Tumour growth curve after the first tumour challenge (10 5 cells) on prophylactically vaccinated mice. ( c ) A comparison of the survival rate in re-challenged mice prophylactically treated with (A) bolus injection (4 × 10 5 irradiated B16-F10 cells+soluble 3 μg GM-CSF+soluble 100 μg CpG ODN); (B) Cryogel vaccine (2 × 2 × 10 5 irradiated B16-F10 cells+2 × 1.5 μg GM-CSF+2 × 50 μg CpG ODN); (D) Cryogel vaccine (2 × 2 × 10 5 irradiated B16-F10 cells+2 × 50 μg CpG ODN); and (F) naive mice (no immunization). At day 126 following immunization, C57BL/6 J mice (10 mice/group) from the first challenge study were challenged a second time with 10 5 B16-F10 tumour cells and monitored for survival. ( d ) Overall survival rate after two consecutive tumour challenges in prophylactically immunized mice to evaluate long-term immunological protection in the context of melanoma. Overall survival is defined as the fraction of mice that survive both challenges. ( e ) A comparison of the survival of mice bearing established melanoma tumours (inoculated with 5 × 10 5 B16-F10 cells and allowed to develop for 3 days, tumour area≥10 mm 2 ) and therapeutically treated with cryogel vaccines (2 × 2 × 10 5 irradiated B16-F10 cells+2 × 1.5 μg GM-CSF+2 × 50 μg CpG ODN) either once at day 3 (Cryogel Vax – 1X) or at both days 3 and 10 (Cryogel Vax – 2X), or naive mice (Control, no immunization). ( f ) Individual tumour growth curves for each mouse surviving tumour challenge (5 × 10 5 cells) after a two-time treatment with cryogel vaccines at days 3 and 10. Values represent mean and s.d. ( n =10 per condition) from at least two independent studies. For simplification, only Fig. 6b shows the legend but it applies also to Fig.6a, c and d. Data were analysed using χ 2 -test, log-rank test (survival curves comparison), or one-way analysis of variance (ANOVA) (** P <0.01, *** P <0.001). Full size image The long-term protective immune response elicited by cryogel vaccinations was next tested. Approximately 4 months following vaccination and subsequent challenge, mice that survived the initial challenge were challenged for a second time. Initial vaccination with the complete cryogel vaccine (GM-CSF, CpG ODN and tumour cells) induced a very strong immunological memory, as 100% of the vaccinated mice that survived the initial challenge survived the second challenge ( Fig. 6c ). Approximately 70% of the animals that initially received cryogel vaccines lacking GM-CSF survived a second challenge. Vaccination with the bolus control group resulted in much lower survival with the second challenge. The data suggest that cryogel vaccines can provide a powerful short and long-term protective immune response. The overall survival rate, the fraction of mice that survived both challenges, was next calculated ( Fig. 6d ). The overall survival of mice vaccinated with the complete cryogel vaccine was 80%. Cryogel vaccines lacking GM-CSF were not as effective in generating a long-term active immunological memory response, as these vaccines resulted in only a 50% overall survival rate, indicating the benefit of providing GM-CSF within the matrix to elicit long-term protection ( Fig. 6c,d ). In addition, the benefit of a three-dimensional (3D) vaccine platform was further demonstrated by the low overall survival rate (less than 20%) in the conditions that used a bolus injection without a cryogel. As a preliminary screen of the safety of the cryogel vaccines, explanted implants and organs were sent for pathological review. In the mice, there was no evidence of pathologic changes in any of the organs, although minimal granulomas were noted at the vaccine site. The absence of toxicity in the liver, kidney or other organs suggests that the scaffold-based vaccines may have minimal systemic adverse effects. Cryogel vaccines induce regression of established melanoma Owing to the strong and durable prophylactic immune response elicited after cryogel vaccination, we next tested the activity of the cryogel vaccines in a B16-F10 therapeutic model. Tumours were established via inoculation of 5 × 10 5 cells, and vaccination was performed 3 days later. Untreated, control tumour-bearing mice had tumours that grew rapidly and only survived up to day 29 ( Fig. 6e , Supplementary Fig. 12b ). Injection with a single dose of the cryogel vaccine at day 3 slightly increased the mean survival time compared with controls, but by day 46 all animals required euthanization. However, boosting with a second dose of the cryogel vaccine on day 10 caused the total regression of tumours in a fraction of the animals ( Fig. 6f , Supplementary Fig. 12b ). Strikingly, 40% of the mice vaccinated and boosted with the cryogel vaccines were free of detectable tumours and survived for more than 100 days. Importantly, complete eradication of established tumours of up to 109 mm 3 in volume was found with this treatment ( Fig. 6f ). In contrast, while mice vaccinated with one or two (cryogel-free) bolus vaccines effectively demonstrated a slowing of tumour growth compared with controls, tumours continued to grow and all the mice required to be euthanized by day 38 ( Fig. 7 ). 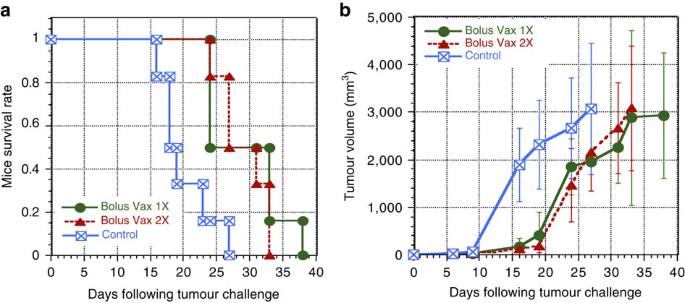Figure 7: Cryogel-free bolus vaccines containing irradiated B16-F10 cells, GM-CSF and CpG ODN confer no therapeutic efficacy. A comparison of the survival (a) and tumour growth (b) of C57BL/6 J mice bearing established melanoma tumours (inoculated with 5 × 105B16-F10 cells and allowed to develop for 3 days, tumour area≥10 mm2, six mice/group) and therapeutically treated with a cryogel-free bolus vaccine (Bolux Vax 1X: 4 × 105irradiated B16-F10 cells+soluble 3 μg GM-CSF+soluble 100 μg CpG ODN) at day 3 or cryogel-free bolus vaccines (Bolux Vax 2X: 4 × 105irradiated B16-F10 cells+soluble 3 μg GM-CSF+soluble 100 μg CpG ODN) at both days 3 and 10; and (Control, no immunization): naive mice. Figure 7: Cryogel-free bolus vaccines containing irradiated B16-F10 cells, GM-CSF and CpG ODN confer no therapeutic efficacy. A comparison of the survival ( a ) and tumour growth ( b ) of C57BL/6 J mice bearing established melanoma tumours (inoculated with 5 × 10 5 B16-F10 cells and allowed to develop for 3 days, tumour area≥10 mm 2 , six mice/group) and therapeutically treated with a cryogel-free bolus vaccine (Bolux Vax 1X: 4 × 10 5 irradiated B16-F10 cells+soluble 3 μg GM-CSF+soluble 100 μg CpG ODN) at day 3 or cryogel-free bolus vaccines (Bolux Vax 2X: 4 × 10 5 irradiated B16-F10 cells+soluble 3 μg GM-CSF+soluble 100 μg CpG ODN) at both days 3 and 10; and (Control, no immunization): naive mice. Full size image A key challenge in cancer vaccine design is to overcome the lack of co-stimulatory signals and presence of tolerogenic signals in the tumour microenvironment, without triggering systemic inflammatory toxicity, thereby extending the clinical scope of cancer vaccines to less immunogenic malignancies. Herein we demonstrate a whole-tumour cell vaccine platform that creates a local immunogenic niche in which the encounter of DCs and tumour cells is tightly controlled, favouring the induction of a potent and durable anti-tumour immune response. The cryogels described in this report were designed to be injected subcutaneously with a standard syringe, which represents a significant advantage over the requirement for surgical implantation of our previously described PLGA scaffold vaccines, while combining the benefits of cell vaccination with those of depot-based formulations by creating an environment to support irradiated tumour cells and infiltrating leukocytes while concomitantly controlling the delivery of recruitment and immunoregulatory factors [19] , [21] . These cryogels can be compressed to a fraction of their original volume and return to their original shape following injection. Within this material the transplanted tumour cells have a high viability immediately following injection, and the cryogels release immunomodulatory factors in a localized and sustained manner, obviating the need for ex vivo genetic manipulation of either the tumour or bystander cells, while in cancer models attaining greater survival rates than bolus administration of the immunoactive factors alone. Unlike strategies that separately deliver adjuvant and antigen, such as the delivery of TLR agonists with CDX-1401 that has found some success in phase 1 trials in refractory malignancies [22] , the cryogel vaccine can be engineered to coordinate the delivery of both adjuvant and antigen in space and time, potentially enhancing overall vaccine performance by more closely matching factor delivery with the kinetics of DC-T-cell priming and activation. Unlike the tolerogenic milieu of the tumour bed or bolus administration of immunoactive factors, the vaccine platform is designed to provide appropriate DC co-stimulation through creating a local space where DCs can interface with tumour cells in the presence of immunomodulatory factors [23] , [24] . Specifically, the macropores create a physical space for DCs and tumour cells to interact in the presence of the released immunomodulatory factors, without the tolerogenic milieu present in the tumour bed. Unlike bolus delivery of tumour cells and adjuvant, the cells and immunomodulatory agents are localized into a small volume, and the delivery of factors in space and time can be quantitatively controlled. As the immunomodulatory factors are released locally, few systemic effects are anticipated, in contrast to systemically delivered agents, such as immune checkpoint blocking antibodies [4] , [25] , [26] , [27] , [28] , [29] , [30] , [31] , [32] , [33] . Still, given the recent success of checkpoint blockade in a variety of cancers, future studies that examine these therapies (or the BRAF/MEK inhibitors) in conjunction with the cancer vaccine platform presented here are warranted [1] , [2] , [3] , [4] , [32] , [34] . Multiple strategies have been used to harness DC to invoke anti-tumour responses including DC adoptive transfer, antibody targeting, biomaterial depots, nanoparticle delivery, and more recently lymph node targeted antigen-adjuvant immunoconjugates [22] , [35] , [36] , [37] , [38] , [39] , [40] , [41] . Many of these approaches have been successful in preclinical and clinical trials and often target lymph node antigen-presenting cells. To date it is not clear which DC population(s) should be targeted for a given malignancy. The cryogel vaccine platform described above targets peripheral dendritic cells and likely can be engineered to potentially allow for both peripheral and central activity. Moreover, unlike the aforementioned strategies, the cryogel vaccine creates a physical space for cell infiltration that we expect limits the effects of deleterious signalling in the microenvironment. Future studies including labelled tumour cells would be valuable to better evaluate both the subtype of DCs and the trafficking of antigen to the draining lymph nodes. Numerous DCs of multiple subtypes are enhanced in the vaccine platform. A total of more than 2 million DCs are recruited locally, comparable to the number of DCs administered in adoptive transfer protocols. Similar to what was observed with other material systems that deliver CpG ODN and GM-CSF, conventional and plasmacytoid DCs were both enriched [18] . Slightly more than 50% of the DCs recruited are of the plasmacytoid type, a subpopulation important for IFN elaboration that is critical for tumour clearance [42] . There is, however, also a substantial fraction of conventional DCs, including a subset of CD8 + DCs capable of antigen cross-presentation, which is thought to be essential in tumour immunity [38] , [43] . Therefore, the spectrum of DCs elicited by the vaccine is larger than the narrow pool of selected DCs typically administered in adoptive transfer [44] , [45] . Further, the local DC numbers remain elevated for many days giving further opportunities to influence DCs fate. This accumulation of DCs is achieved both by delivering GM-CSF from the cryogel system and by creating macropores that facilitate cellular infiltration and trafficking. Importantly, the DCs accumulate in situ and are thus likely not susceptible to the loss in cell function and number observed during typical adoptive transfer, nor do they require ex vivo pulsation with tumour antigens or treatment with maturation factors [46] , [47] , [48] , [49] . Also, in comparison with GVAX or FVAX, no additional ex vivo genetic manipulation of transplanted tumour cells is required. This diversity of DCs is reflected in the local cytokine profile, which includes both Th1 associated (IL-2) and Th2 associated (IL-13, IL-10) cytokines in addition to a multitude of strong pro-inflammatory factors (RANTES, Eotaxin, IL-1b, GM-CSF, MCP-1b and MCP-1a among others). Surprisingly, no statistically significant difference in IL-12 and IFN-γ concentration was observed, and the concentration of these factors was less pronounced than anticipated. As these results were obtained at day 13 when DC numbers are falling, and previous studies have shown an earlier increase followed by a decrease in IL-12 and IFN-γ around this time point, we speculate that at earlier times more substantial IL-12 and IFN signalling may be observed and that perhaps some autoregulation or negative feedback is occurring at the later time points [50] . Similarly, these results are obtained more proximally from the vaccination site. Although less central to the hypothesis of this work, it would be interesting to probe the cellular and cytokine profile in more depth more downstream at the level of the draining lymph node. The injectable cryogels elicit a potent and durable immune response. Over 3.5 million T cells including CTLs are recruited locally, though the antigenic specificity of these remains to be clarified. The enhancement in CTLs is associated with a rise in the ratio of CD8 + to FoxP3 + cells, indicating the enhancement of protective immunity and a reduction in immunosuppressive mechanisms. The rise in effector T cells coincides with durable protection in both prophylactic and therapeutic models of B16-F10 melanomas building upon previous GVAX studies and biomaterial vaccination approaches [2] , [3] , [51] . Although, the response of cytotoxic and helper T cells was explored, the role of melanoma-specific CD8 + T cells was not investigated. Similar to previous studies, we anticipate the cryogel system to trigger large numbers of TRP2-specific CD8 + T cells following vaccination of mice [18] . Still, there is a possibility that other antigens against other types of cancer cells may be eliciting the potent immunoprotection observed in this study. It remains to be examined whether alternative arms (for example, humoral arm) and cell mediators of the immune system are partially responsible for the findings reported here, and further investigations are warranted. The overall enhancement of animal survival is most notably observed in the therapeutic model. In the B16 murine melanoma model it is well known that vaccination strategies that are efficacious in the prophylactic model often fail in the therapeutic setting [52] . In the work described herein, this is most notably observed in the difference between the bolus delivery group and the cryogel vaccination group. These discrepancies could reflect different underlying mechanisms of action between the two delivery approaches; however, they more likely reflect different overall potencies between the two vaccination strategies. Further, the therapeutic strategy is more reflective of the actual clinical scenario where these vaccines would be used and in this setting is where the cryogel demonstrates its greatest efficacy in comparison with other vaccination approaches. Still, the B16 model is one preclinical melanoma model and differences exist between preclinical and clinical models and further testing should be pursued [53] . One limitation of this vaccination approach is the requirement for tumour cells. However, minimal manipulation of these cells is required ex vivo and the use of whole tumour cells provides a wide breadth of tumour antigens. Isolating sufficient cell numbers can be a problem for autologous tumour cell vaccines, and future studies will evaluate whether the number of tumour cells needed for effective vaccination can be reduced with this system [13] . Given that a large number of cells die or lose function during manipulation and that some of the losses can be mitigated with the use of material systems, the cryogel system may represent a significant improvement over more traditional cell-based vaccine approaches [54] . Recently, adoptive transfer of tumour-infiltrating lymphocytes was shown to induce regression for a subset of patients with carcinomas, the most prevalent solid tumours [55] . The strategy described herein could potentially be completed in parallel with similar T-cell adoptive transfer techniques and raises the question of whether T-cell selection and expansion could occur in situ within the vaccine platforms. In addition to vaccination against melanoma, this strategy may also be applicable to other types of cancer, and studies are ongoing testing this platform in additional cancer models. More broadly, this platform may be useful for generating a range of T-effector responses from immunity to tolerance. For example, mesenchymal stem cells could be loaded onto the platform and delivered to elicit tolerogenic type responses in the setting of autoimmunity or transplantation. Materials UP LVG sodium alginate with high guluronate content was purchased from ProNova Biomedical; 2-morpholinoethanesulfonic acid (MES), sodium chloride (NaCl), calcium chloride (CaCl 2 ) sodium hydroxide (NaOH), N- hydroxysuccinimide (NHS), 1-ethyl-3-(3-dimethylaminopropyl)-carbodiimide hydrochloride (EDC), 2-aminoethyl methacrylate hydrochloride (AEMA) and acetone were purchased from Sigma-Aldrich. ACRL-PEG-NHS (3.5 kDa) was purchased from JenKen Technology. Rhodamine-labelled polylysine was obtained from Nanocs. Alexa Fluor 488-phalloidin and 4',6-diamidino-2-phenylindole (DAPI) were purchased from Life Technologies. The integrin binding peptide (Gly) 4 -Arg-Gly-Asp-Ala-Ser-Ser-Lys-Tyr (G 4 RGDASSKY) was custom made by Commonwealth Biotech. Wild-type B16-F10 cells (ATCC) were cultured in Dulbecco’s modified Eagle medium (DMEM) supplemented with 10% (vol/vol) FBS and 1% (vol/vol) penicillin–streptomycin, all obtained from Invitrogen [9] . Cryogel vaccine fabrication First, methacrylated alginate (MA-alginate) was prepared by reacting alginate with AEMA. Sodium alginate (1 g) was dissolved in a buffer solution (0.6% (wt/vol), pH ∼ 6.5) of 100 mM MES. NHS (1.3 g) and EDC (2.8 g) were added to the mixture to activate the carboxylic acid groups of alginate. After 5 min, AEMA (2.24 g; molar ratio of NHS:EDC:AEMA=1:1.3:1.1) was added to the product and the solution was stirred at room temperature (RT) for 24 h. The mixture was precipitated in acetone, filtered and dried in a vacuum oven overnight at RT. 1 H NMR was used to characterize chemical modification of alginate and degree of functionalization of MA-alginate ( Supplementary Fig. 13 ). Macroporous matrices were synthesized by redox-induced free-radical polymerization of MA-alginate in deionized water. ACRL-PEG-G 4 RGDASSKY was synthesized by coupling amine-terminated G 4 RGDASSKY peptide to an acrylate-PEG-N-hydroxysuccinimide comonomer [16] . Alginate cryogel vaccines were synthesized by mixing 23 mg (2.3% (wt/vol)) of MA-alginate macromonomer per ml of deionized water with tetramethylethylenediamine (TEMED) (0.5% (wt/vol)) and ammonium persulfate (APS) (0.25% (wt/vol)). CpG ODN 1826, 5′-TCC ATG ACG TTC CTG ACG TT-3′ (Invivogen), and GM-CSF (PeproTech) were added to the polymer solution before cryopolymerization. Fabrication conditions were chosen to allow the solution to freeze before the gelation takes place. More specifically, the precursor solution was precooled to 4 °C to decrease the rate of polymerization before freezing, and once the initiator was added to the prepolymer solution, the solution was quickly poured into a precooled (−20 °C) Teflon mold. After a complete incubation period of 17 h, the gels were heated to RT to remove ice crystals and washed with deionized water. Cell-adhesive cryogels were synthesized using ACRL-PEG-G 4 RGDASSKY as a comonomer (0.8% (wt/vol)) during the polymerization. Conventional hydrogels were cross-linked for 30 min at RT for a homogeneous gelation. Cell seeding and incubation of cellular cryogel vaccines Before seeding cells, the cryogels were treated with 70% ethanol and washed with PBS. The cryogels were mechanically compressed to partially remove pore water under sterile conditions before cell seeding. Before seeding, the B16-F10 cells were irradiated by receiving 3,500 rads (1 rad=0.01 Gy) from a 137Cs source discharging 208 rads min −1 for 17 min. Twenty microliters of a cell suspension (10 7 cells ml −1 ) in complete culture medium (DMEM supplemented with 10% FBS and 1% penicillin–streptomycin) were added in a dropwise manner on top of each square-shaped cryogel and the cell-loaded cryogels were cultured in FBS-supplemented media for 6 h (37 °C in 5% CO 2 environment). Cell distribution was noted to be homogeneous throughout the gel construct. Controlled release of immunodulator factors To determine the incorporation efficiency and release kinetics of CpG ODN and GM-CSF from cryogel vaccines, gels were incubated in sterile PBS at 37 °C with shaking. Samples were withdrawn periodically and replaced with the same amount of fresh PBS. GM-CSF and CpG ODN released in the supernatant were detected by ELISA (Invitrogen) and OliGreen assay (Invitrogen), respectively. Bioactivity of released GM-CSF The fraction of bioactive GM-CSF released from the cryogels was assessed by an in vitro bioactivity assay. Bone marrow cells were isolated from C57BL/6 J mice (female, aged 6-8 weeks; Jackson Laboratories). A total of 4 × 10 4 cells in 100 μl of RPMI-1640 media (supplemented with 10% heat-inactivated FBS, 1% penicillin/streptomycin, 50 uM β-mercaptoethanol) were seeded in each well of black tissue culture treated 96-well plates. A 7-point standard curve was prepared by performing fourfold serial dilutions of a 40 ng ml −1 GM-CSF solution in HBSS (containing 1% BSA and 1% penicillin/streptomycin). To each well, 100 μl of samples, standards or a blank control were added, in triplicate, and cells were cultured at 37 °C for 5 days. 10% v/v of AlamarBlue reagent (Life Technologies) was added to each well, and after a 4-h incubation at 37 °C, plates were read on a BioTek plate reader to measure the absorbance at 490 nm. All standards and samples were normalized to the blank controls, and the bioactivity of the experimental samples was determined relative to the standard curve. ‘% bioactivity’ was calculated by normalizing the amount of GM-CSF bioactivity to the amount of GM-CSF protein detected by ELISA for the same sample. Hydrogel characterization Structural analysis of the macroporous gel-vaccine was performed using a LEO 982 scanning electron microscope (s.e.m.) (LEO Electron Microscopy). To prepare the samples, cryogels in the frozen state following cryogelation were lyophilized and sectioned for observation. The average size of pores in cryogels was calculated by averaging the diameters of the pores in the gels observed by s.e.m. The distribution of cells within the scaffolds was visualized with an inverted laser scanning confocal microscope (Leica SP5 XMP, Germany). High-resolution image stacks were collected with 300-nm separation between slices (z-stacks) for the 3D reconstruction of the entire scaffold and visualization of cell–matrix interactions. Generation of BMDCs and in vitro DCs activation assays Bone marrow-derived DCs (BMDCs) were generated from isolated murine hindlimb bones, which were placed in 70% ethanol for 2 min and then washed in PBS [56] . Both distal bone ends were excised and the marrow was flushed with RPMI 1,640 medium (Gibco, Grand Island, NY). The red blood cells were lysed with ammonium chloride (0.45 M). The remaining cells were centrifuged for 10 min at 1,500 r.p.m. and 2 × 10 5 ml −1 cells were aliquoted into Petri dishes in 10 ml of R10 medium (RPMI 1,640 medium supplemented with 10% heat-inactivated FBS, 1% penicillin–streptomycin, 2 mM L -glutamine, 50 μM 2-mercaptoethanol and 20 ng ml −1 murine GM-CSF). On day 3, 10 ml of additional media was added to the plates. On days 6 and 8, 10 ml of media was gently aspirated from the wells, centrifuged down, and to the pellet 10 ml of fresh media was added before re-plating. On day 10 the procedure was repeated, except that media with 10 ng ml −1 of GM-CSF was added. Typical purity was >85% as observed with flow cytometry staining with allophycocyanin (APC)-conjugated CD11c (eBioscience 17-0114, 2.5 μg ml −1 ). To evaluate viability and activation/induction of BMDCs exposed to CpG ODN-loaded cryogel vaccines, square-shaped blank scaffolds or scaffolds containing CpG ODN 1826 (5′ -TCC ATG ACG TTC CTG ACG TT-3′) were incubated with bone marrow DCs in complete culture medium for 1 day (RPMI 1,640 medium supplemented with 10% FBS and 1% penicillin–streptomycin). A live/dead assay was performed to evaluate BMDCs viability in the presence of cryogels. In brief, isolated BMDCs in triplicate were incubated with the live/dead assay dye solution (Molecular Probes) containing 0.5 μl of calcein AM and 2 μl of ethidium homodimer-1 in 1 ml of PBS. After 30-min incubation, the cells were rinsed with PBS, and cell viability was quantified by flow cytometry (FACS). BMDCs maturation was evaluated by flow cytometry using the following antibodies conjugated to fluorescent markers (2.5 μg ml −1 ) for surface stainings: phycoerythrin (PE)-conjugated MHCII (eBioscience 12-5,322), fluorescein isothiocyanate (FITC)-conjugated CD86 (eBioscience 11-0862), APC–conjugated CD11c (eBioscience 17-0114). For purified antibodies the appropriate anti-TNP isotype controls were used. The concentrations of IL-6, IL-12, and TNF-α in the cell-culture supernatant were then analysed with ELISA (R&D systems), according to the manufacturer’s instructions. Delivery of cryogel cancer vaccines and cell recruitment Female BALB/c or C57BL/6 J mice ( n =8; The Jackson Laboratory), 6–8 weeks of age, were anaesthetized with 2.5% isoflurane using an inhalation anaesthesia system (E-Z Anaesthesia; Euthanex). Each mouse received subcutaneous injections of two cryogels (alternatively, cryogels were implanted when non-injectable nanoporous hydrogels were used as a control in one experiment) suspended in 0.2 ml of sterile PBS into the dorsal flank by means of a 16-gauge needle. To visualize the cell-recruitment and homing capacity of cryogels, mice were euthanized 4 days post-injection, and the explanted scaffolds were embedded in paraffin and 5-μm sections were stained with haematoxylin and eosin (H&E) for histological analysis. Alternatively, to quantify dendritic cell recruitment, explanted cryogels were digested in collagenase type II (250 U ml −1 ; Worthington) that was agitated at 37 °C for 45 min. The cell suspensions were then poured through a 40-μm cell strainer to isolate cells from scaffold particles, and the cells were pelleted and washed with cold PBS and counted with a Z2 coulter counter (Beckman Coulter). To assess DC infiltration, cells isolated from alginate sponges were then stained with primary antibodies conjugated to fluorescent markers (2.5 μg ml −1 ) to allow for analysis by flow cytometry. Specifically, APC-conjugated CD11c (eBioscience 17-0114) staining was conducted to analyse for DC infiltration. Unless stated otherwise, for all flow cytomety studies cells were gated based on forward and side-scatter characteristics to limit debris including dead cells. Animal work was performed under a protocol approved by the Harvard Standing Committee on Animals in compliance with the National Institutes of Health guidelines. In situ identification of DC subsets and T cells Two blank alginate cryogel sponges or two cryogel sponges containing 1.5 μg/cryogel of GM-CSF in combination with 50 μg/cryogel of CpG ODN were injected subcutaneously into the dorsal flank of 6- to 8-week-old female C57BL/6 J mice. At various time points, explanted scaffolds, spleens, and LN were digested and isolated cells analysed. To assess DC infiltration and activation, subsets of the total cell population were stained with primary antibodies (2.5 μg ml −1 ) conjugated to fluorescent markers to allow for analysis by flow cytometry. APC-conjugated CD11c (DC marker, eBioscience 17-0114) and PE-conjugated CD86 (B7 costimulatory molecule, eBioscience 12-0862) stains were conducted for DC recruitment analysis, and APC-conjugated CD11c and PE-conjugated MHCII (eBioscience 12-5322) stains were conducted for DC activation analysis. To further delineate the presence of specific DC subsets, cells were stained with APC-conjugated CD11c and PE-conjugated PDCA-1 (pDC marker, eBioscience 12-3171), APC-conjugated CD11c and PE-conjugated CD8 (CD8 DCs, eBioscience 12-0081), or APC-conjugated CD11c and FITC-conjugated CD11b (CD11b DCs, eBioscience 11-0112). To assess T-cell infiltration, PE-Cy7-conjugated CD3 (eBioscience 25-0031) stains in conjunction with APC-conjugated CD8a (CD8 T cells, eBioscience 17-0081), FITC-conjugated CD4 (CD4 T cells, eBioscience 11-0041) and PE-conjugated FoxP3 (Treg, eBioscience 12-5773) were performed and immunofluorescently labelled cells were analysed with flow cytometry. Cells were gated according to positive FITC, APC and PE with isotype controls, and the percentage of cells staining positive for each surface antigen was recorded. To determine the concentration of different cytokines at the cryogel vaccine site, adjacent tissue was excised and digested with tissue protein extraction reagent (Pierce). Cytokine concentrations in the tissue were then analysed with a Bio-Plex Pro Mouse Cytokines 23-plex Immunoassay (Bio-Rad M60009RDPD), according to the manufacturer’s instructions. The Bio-plex was normalized over the amount of tissue extracted. Prophylactic and therapeutic efficacy Two square-shaped RGD-containing alginate sponges pre-cultured with irradiated B16-F10 melanoma cells (ATCC, tumour cells cultured in DMEM supplemented with 10% FBS and 1% penicillin–streptomycin at 37 °C in 5% CO 2 environment). Two gels, each seeded with 2 × 10 5 cells and each loaded with GM-CSF (1.5 μg) and CpG ODN (50 μg) were subcutaneously injected in PBS (0.2 ml/gel) into each side of the lower flank of C57BL/6 J mice ( n =10/group, in vivo experiment performed twice) (Group B, vaccine of interest). For control groups, mice were also injected with two tumour cell-seeded (2 × 10 5 ) blank alginate sponges or with two tumour cell-seeded (2 × 10 5 ) sponges loaded with one single immunomodulatory factor, either GM-CSF (1.5 μg) or CpG ODN (50 μg) (Groups E, C and D, respectively). One control group of mice was vaccinated with a cryogel-free (bolus) vaccine combining both 5 × 10 5 irradiated (3,500 rads) B16-F10 cells and soluble immunomodulatory factors (3 μg GM-CSF and 100 μg CpG ODN) (Group A). Animals were challenged 6 days later with a subcutaneous injection of 10 5 B16-F10 melanoma cells in the back of the neck. To assess long-term immunological response to melanoma vaccines, surviving mice in each groups (A:6, B:8, D:7) and a new set of untreated mice (control, F:10) were re-challenged 126 days following the first tumour challenge with 10 5 B16-F10 melanoma cells. Animals were monitored for the onset of tumour growth (approximately 1 mm 3 ) and euthanized for humane reasons when challenge tumours reached 20 mm (longest diameter) or severe ulceration or bleeding developed. Following 18 months after initial tumour challenge, surviving immunized mice from successive tumour inoculations (days 6 and 126 post vaccination) were euthanized and their tissues evaluated for evidence of toxicity. Tissues from the major organs (the heart, liver, spleen, lungs, kidney, brain, lymph nodes, pancreas, small intestine, colon and stomach) and explanted implants were fixed in a 10% neutral buffered formalin solution, resuspended in 70% ethanol and analysed by Mass Histology Service (Worcester, MA) for toxicology. To assess cryogel vaccine efficacy in the therapeutic setting, C57BL/6 J mice ( n =10/group, in vivo experiment performed twice) were challenged with a subcutaneous injection of 5 × 10 5 B16-F10 cells into the nape of the neck. At day 3 after tumour challenge, two square-shaped cryogel vaccines loaded with GM-CSF (1.5 μg/cryogel), CpG ODN (50 μg/cryogel) and irradiated B16-F10 melanoma cells (2 × 10 5 cells/cryogel) were injected subcutaneously into the lower flank of C57BL/6 J mice. A subset of mice was vaccinated again at 10 days after the initial tumour cell challenge. Statistical analysis All values in the present study were expressed as mean±s.d. The significance of differences between the groups was analysed by a Student’s t -test, one-way analysis of variance (ANOVA) with Tukey or Bonferroni post hoc analysis, χ 2 -test, or a log-rank test was used to compare two or more groups of survival times depending on their relevance for each comparison. Differences were considered significant at P <0.05. How to cite this article: Bencherif, S. A. et al . Injectable cryogel-based whole-cell cancer vaccines. Nat. Commun. 6:7556 doi: 10.1038/ncomms8556 (2015).